Enantioselective reduction of sulfur-containing cyclic imines through biocatalysis The 3-thiazolidine ring represents an important structural motif in life sciences molecules. However, up to now reduction of 3-thiazolines as an attractive approach failed by means of nearly all chemical reduction technologies for imines. Thus, the development of an efficient general and enantioselective synthetic technology giving access to a range of such heterocycles remained a challenge. Here we present a method enabling the reduction of 3-thiazolines with high conversion and high to excellent enantioselectivity (at least 96% and up to 99% enantiomeric excess). This technology is based on the use of imine reductases as catalysts, has a broad substrate range, and is also applied successfully to other sulfur-containing heterocyclic imines such as 2H -1,4-benzothiazines. Moreover the effiency of this biocatalytic technology platform is demonstrated in an initial process development leading to 99% conversion and 99% enantiomeric excess at a substrate loading of 18 g/L in the presence of designer cells. Cyclic amines with a sulfur-atom in the heterocyclic structure play a distinguished role in nature and medicine. In particular, this is true for the 3-thiazolidine ring, which is one of the two heterocyclic framework structures present in penicillins and penicillin-derived β-lactam antibiotic drugs such as amoxicillin [1] . The 3-thiazolidine moiety is also a structural motif in a range of HIV protease inhibitors [2] and an industrial key intermediate for the production of the non-proteinogenic amino acid d -penicillamine [3] (Fig. 1 ). In addition, spiro -type 3-thiazolidines showed activity in human tumor cell lines [4] , and 3-thiazolidines with a less functionalized, alkyl-substitution pattern are of pharmaceutical interest with applications, e.g., as radioprotective agents [5] , [6] . Besides medicinal purpose, alkyl-functionalized 3-thiazolidines are reported to be relevant for the fields of pesticides [7] and flavors [8] (Fig. 1 ). Due to the importance of such molecules and the lack of efficient general synthetic approaches, the search for attractive synthetic routes towards 3-thiazolidines (and other pharmaceutically interesting sulfur-containing cyclic amines such as 3,4-dihydro-2 H -1,4-benzothiazines [9] ) is still ongoing. The development of a general and enantioselective synthetic platform technology giving access to a broad range of such heterocycles independent of a specific substitution pattern, thus enabling the design of libraries of such heterocycles, as well as efficient processes for their production, would be particularly desirable. Fig. 1 Application areas of 3-thiazolidines. Examples for pharmaceutical relevant structures containing 3-thiazolidines as structural moiety Full size image Conceptually a substitution pattern independent access towards 3-thiazolidines 2 can be proposed to proceed through reduction of the C=N double bond in the corresponding 3-thiazolines ( 1 ), which can be easily prepared through Asinger-type multicomponent reaction [10] , [11] , [12] , [13] . However, in spite of the availability of such attractive substrates, in all research work since the 1950s the reduction of 3-thiazolines ( 1 ) failed by means of nearly all state of the art-type chemical reduction technologies for imines. Such non-successful attempts include numerous typical C = N double bond reduction technologies, which are known to work well for many other imine substrate types. For example, the established hydrogenation technology (Pd/C, H 2 ) was found at an early stage not to be suitable due to catalyst poisoning by sulfur [13] , [14] . These results are in accordance with later results by the Figueras group, finding that metals of supported metal catalysts become poisoned by sulfur [15] . The recently developed organocatalytic reduction with Hantzsch esters for imines [16] , [17] also failed to lead the desired transformation due to lack of reactivity (Supplementary Figs. 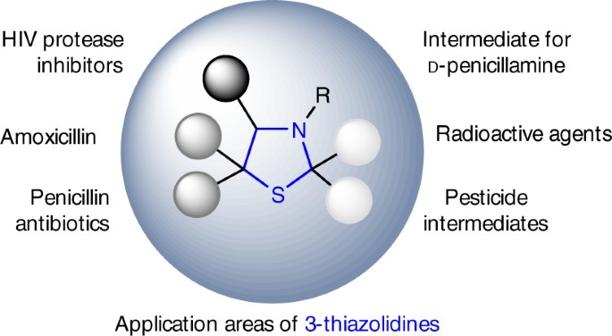Fig. 1 Application areas of 3-thiazolidines. Examples for pharmaceutical relevant structures containing 3-thiazolidines as structural moiety 1 , 2 , Supplementary Table 1 and Supplementary Methods). Other well-established reduction methods, such as sodium in alcohol, sodium in liquid ammonia or aluminum in the presence of potassium hydroxide or wet ether did not give clear results [13] . When using metal hydrids, such as NaBH 4 and LiAlH 4 , reduction works but is accompanied with an undesired ring-opening of the N , S -acetal moiety in the product 2 (Supplementary Fig. 2 and Supplementary Methods) [13] , [14] , [18] . The only exception is a catecholborane-type reduction [18] , but in this case the yield was low to moderate and enantioselectivity turned out to be poor with only up to 4% enantiomeric excess (ee). In addition, a high-catalyst loading, as well as an expensive and technically less favored reducing agent (due to high flammability) is needed. Thus, the development of an efficient general method for the reduction of 3-thiazolines ( 1 ) remained a challenge, as did establishing an asymmetric catalytic version of this reaction. Attracted by the recent successful use of imine reductases (IREDs) for various reductions of cyclic imines [19] , [20] , [21] , [22] , [23] , [24] , [25] , [26] , [27] , [28] , [29] , [30] , we became interested in studying the suitability of this biocatalytic methodology for the reduction of 3-thiazolines ( 1 ) and other sulfur-containing cyclic imines such as 2 H -1,4-benzothiazines ( 3 ). Here we report such a biocatalytic reduction which firstly enables a smooth reduction of 3-thiazolines ( 1 ) avoiding undesired ring-opening or other side reactions, secondly allows a highly enantioselective synthesis of the resulting 3-thiazolidines ( 2 ) by means of such an approach starting from 3-thiazolines ( 1 ), and thirdly is a broadly applicable reduction platform for sulfur-containing heterocyclic imines including 3-thiazolines ( 1 ), as well as other sulfur-containing heterocyclic imines such as 2 H -1,4-benzothiazines ( 3 ). Proof of concept for 3-thiazoline reduction In initial experiments, we tested whether IREDs are suitable biocatalysts for the reduction of 3-thiazolines (Fig. 2 ). Although unknown for cyclic imines with additional heteroatoms, we focused on this enzyme class instead of the so-called thiazolinyl IREDs since the latter enzymes (although bearing the term thiazolinyl imine in their name) are known to be substrate-specific for structurally highly functionalized 2-thiazolines reducing an imidothioester moiety [31] , [32] , thus representing no promising option for developing a broadly applicable synthetic platform for the reduction of the imine bond of 3-thiazolines. Toward this end, we prepared two non-prochiral 3-thiazolines ( 1a and 1b ) and screened them against a set of 31 IREDs, which had been prepared in a recombinant form by means of overexpression in E . coli BL21 (DE3) [22] , [29] . As a fast screening methodology a colorimetric pH shift assay [33] developed by the Sieber group was used. This assay is based on a pH shift (visualized by bromthymol blue), which is caused by gluconic acid formed by consumption of the substrate and in situ-cofactor-regeneration (Fig. 3 , Supplementary Figs. 3 , 4 and Supplementary Methods). Fig. 2 Concept of this work. a Access toward 3-thiazolines via Asinger-type synthesis and subsequent reduction to 3-thiazolidines. Whereas nearly all classic chemical and chemocatalytic approaches toward reduction of 3-thiazolines failed, reduction with imine reductases provided 3-thiazolidines in high conversion and enantioselectivity. b The biocatalytic approach using imine reductases was also successfully applied for the reduction of other sulfur-containing heterocyclic imines, such as 2 H -1,4-benzothiazines Full size image Fig. 3 Colorimetric pH shift assay of 3-thiazolines. a Concept of colorimetric pH shift assay. Reduction of substrate catalyzed by imine reductase (IRED) and in situ-cofactor-regeneration by glucose dehydrogenase (GDH) results in a pH shift, due to formation of gluconic acid. This pH shift is visualized by bromthymol blue as indicator. 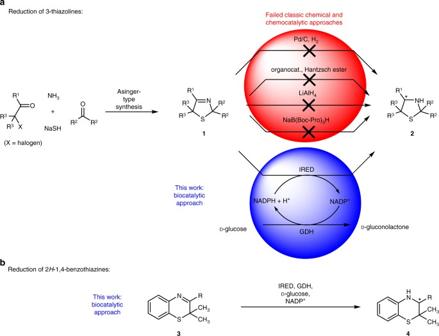Fig. 2 Concept of this work.aAccess toward 3-thiazolines via Asinger-type synthesis and subsequent reduction to 3-thiazolidines. Whereas nearly all classic chemical and chemocatalytic approaches toward reduction of 3-thiazolines failed, reduction with imine reductases provided 3-thiazolidines in high conversion and enantioselectivity.bThe biocatalytic approach using imine reductases was also successfully applied for the reduction of other sulfur-containing heterocyclic imines, such as 2H-1,4-benzothiazines b Substrate spectrum of 3-thiazolines examined in this work Full size image Color changes from green to yellow were observed for both non-prochiral 3-thiazolines 1a and 1b in combination with a range of IREDs (Supplementary Table 2 ). Negative controls without an IRED showed no color change, indicating that the utilized glucose dehydrogenase (GDH) has no side-activity toward such an imine reduction (in contrast to analogous reductions of other imines as reported in ref. [34] ). We subsequently performed biotransformations at a substrate concentration of 20 mM of 3-thiazoline 1b using two IREDs, which were prioritized according to the results from the colorimetric pH shift assay. For in situ-cofactor regeneration, once again a GDH from Bacillus subtilis [25] , [35] was used in combination with d -glucose as a co-substrate. After a reaction time of 24 h, formation of 3-thiazolidine 2b was demonstrated (Table 1 , entry 1), and revealed conversions of 29 and 83% with perfect product selectivity even under non-optimized reaction conditions. Thus, these results demonstrate that IREDs are suitable biocatalysts for the reduction of 3-thiazolines avoiding undesired ring-opening or other side reactions known for classic chemical and chemocatalytic reduction methodologies. Table 1 Reduction of 3-thiazolines using imine reductases (IREDs) Full size table Investigation of 3-thiazolines Next, we focused on the study of the substrate scope, as well as the determination of the enantioselectivity of these IRED-catalyzed reduction of 3-thiazolines. Toward this end, we prepared a range of prochiral 3-thiazolines 1c – 1f , comprising monocyclic and spiro -type compounds (Fig. 3 b and Table 1 ). Based on the results of the colorimetric pH shift assay for these 3-thiazolines (Supplementary Fig. 4 and Supplementary Table 2 ), the specific activities were determined by means of a spectrophotometric study, and it is noteworthy that activities were found for all studied 3-thiazolines (Supplementary Figs. 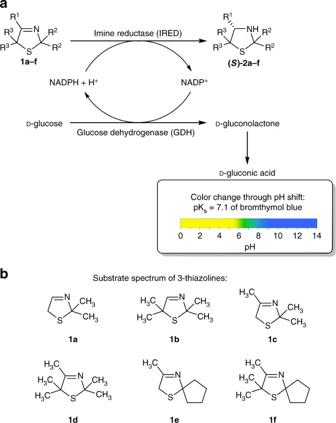Fig. 3 Colorimetric pH shift assay of 3-thiazolines.aConcept of colorimetric pH shift assay. Reduction of substrate catalyzed by imine reductase (IRED) and in situ-cofactor-regeneration by glucose dehydrogenase (GDH) results in a pH shift, due to formation of gluconic acid. This pH shift is visualized by bromthymol blue as indicator.bSubstrate spectrum of 3-thiazolines examined in this work 5 , 6 and Supplementary Table 3 ). Utilizing the IREDs which showed the highest specific activities, biotransformations of the prochiral 3-thiazolines running at a 20 mM substrate concentration on a 10 mL scale and in situ-cofactor regeneration with a GDH were performed (Table 1 , entry 2–5). We found that for each substrate at least one IRED catalyzes the reduction with good to excellent conversion (82–98%) under non-optimized reaction conditions (Table 1 ). Activity was higher when R 3 comprises methyl groups as substituents compared to the sterically less hindered hydrogen. Thus, when starting from prochiral 3-thiazolines 1c and 1e , which bear hydrogens at R 3 , a higher total protein concentration of 5 mg mL −1 had to be used for achieving good conversions (Table 1 , entry 2, 4). In contrast, for good to excellent conversions a much lower amount of IRED8 [22] with a total protein concentration (crude extract) of 1.2 mg mL −1 was sufficient when utilizing prochiral 3-thiazolines 1d and 1f (Table 1 , entry 3, 5). Moreover, a higher activity of IRED8 [22] as well as conversion was found when using spiro -cyclic 3-thiazolidine 1e and 1f compared to the analogous 3-thiazolidines bearing methyl groups as substituents R 2 , 1c and 1d . The highest activity of all tested 3-thiazolines could be determined with the spiro -cyclic compound 1f , which supports our observation that methyl groups at R 3 , as well as a spiro -cyclic scaffold as R 2 substituents represent the best substitution pattern for reduction of 3-thiazolines using IREDs. Negative controls of biotransformations of 3-thiazolines without IRED again showed no conversion, indicating that the utilized GDH has no side-activity towards this imine reduction. Furthermore, we found that IREDs catalyze the reduction of prochiral 3-thiazolines 1c – 1f with high to excellent enantioselectivities (96–99% ee) independent of the substituents R 2 and R 3 (Table 1 , entry 2–5), thus representing the first access to 3-thiazolidines with high-enantiomeric excess via reduction of the C = N double bond in 3-thiazolines ( 1 ). The absolute configuration of the predominant formation of the enantiomers of 3-thiazolidines turned out to be S (section Determination of the absolute configuration of 2f and Table 1 ), which is in accordance with the previously reported selectivity of the imine reducases IRED8 and IRED24 [22] , [29] . The opportunity to reduce monocyclic, as well as spiro -cyclic 3-thiazolines with high conversion and enantioselectivity underlines the value of this biocatalytic approach. Spiro -cyclic scaffolds represent important structural motifs in medicinal chemistry [36] , [37] so that in the future this methodology could be useful toward drug discovery by constructing libraries with structurally highly diverse sulfur-containing spiro -heterocyclic amines. Determination of the absolute configuration of 2f Due to the lack of availability of enantiomerically pure reference compounds (indicating the difficulty to access them by other synthetic methods), we decided to determine the absolute configuration of 2f (obtained from the experiment at elevated lab scale as described in section Process development on 3-thiazoline reduction) by vibrational circular dichroism (VCD) spectroscopy. The experimental IR and VCD spectra of 2f were recorded in choloroform and are shown in Fig. 4 a (for details, see Supplementary Methods). In order to simulate the spectra for the assignment of the configuration, a conformational analysis was carried out first for ( S )- 2f at the MMFF level of theory using Spartan 14 software (Spartan 14, Wavefunction Inc., Irvine, CA, USA (2014)). Subsequently, all eight obtained conformers were subjected to further geometry optimizations followed by spectra calculations at the B3LYP/6-311g++ (2d,p)/IEFPCM(CHCl 3 ) level of theory (using the software Gaussian 09 Rev. E01, Frisch, M.J. et al. Gaussian, Inc., Wallingford CT, USA, (2013)). The relative Gibbs free energies Δ G 298 K and the corresponding Boltzmann weights of the two populated conformers are shown in Fig. 4 b. Based on the single-conformer spectra, the IR and VCD spectra were simulated by assigning a Lorentzian band shape to the dipole and rotational strength calculated for each conformer and subsequent Boltzmann-averaging of the spectra. Direct comparison of the resulting simulated IR and VCD spectra with the experimental data, as indicated by the assignments given in Fig. 4 a, reveals a very good agreement. Therefore, the absolute configuration can be assigned with very high confidence as ( S )- 2f . Fig. 4 Determination of absolute configuration of 2f . a Comparison of the experimental and calculated IR and VCD spectra of ( S )- 2f (numbers indicate some characteristic band assignments). b Structures of the two main conformers of ( S )- 2f , corresponding relative Gibbs free energies Δ G 298 K and the corresponding Boltzmann weights Full size image Reduction of 2H -1,4-benzothiazines Afterwards we studied further reductions using other sulfur-containing heterocyclic imines such as 2H -1,4-benzothiazines ( 3 ) as substrates (Fig. 5 ), which have already been chemocatalytically reduced in an asymmetric fashion [16] , [17] , [38] . Therefore, the 2H -1,4-benzothiazines 3a – 3c were prepared. Among these compounds, the prochiral representatives 3b and 3c contain either a methyl or phenyl group as substituents at R (Table 2 ). Again the colorimetric pH shift assay and subsequent spectrophotometric determination of the enzyme activities were conducted and the most promising IREDs prioritized (Supplementary Figs. 3 , 5 , 7 and Supplementary Tables 2 , 3 ). It turned out that the specific activity for 2H -1,4-benzothiazines 3a and 3b were about 10-fold higher compared to those for 3-thiazoline 1f , which showed the highest activity of all tested 3-thiazolines. Moreover, the specific activities for prochiral 2H -1,4-benzothiazine 3c , bearing a phenyl as substituent at the prochiral carbon atom, is also about 10-fold higher compared to the 3-thiazolines 1a-e (Supplementary Figs. 6 , 7 and Supplementary Table 3 ). Based on these encouraging enzyme activities, showing high activity for 2 H -1,4-benzothiazines also with sterically demanding substituents, as a next step synthetic biotransformations were carried out which also enabled us to gain insight into the enantioselectivity of such reactions (Table 2 ). These biocatalytic reductions were conducted at substrate concentrations of 20 mM on a 0.5 mL scale and the cofactor NADPH was recycled in situ by means of a GDH and d -glucose (Fig. 5 ). Fig. 5 Imine reductase-catalyzed reduction of 2 H -1,4-benzothiazines Full size image Table 2 Reduction of 2 H -1,4-benzothiazines using imine reductases (IREDs) Full size table Under non-optimized reaction conditions all 2H -1,4-benzothiazines were converted to the corresponding 3,4-dihydro- 2H -1,4-benzothiazines with moderate to good conversions of up to >99%, and most IREDs turned out to be suitable for catalyzing these reactions. In accordance with the determined enzyme activities, the amount of biocatalyst needed for the reduction of 2H -1,4-benzothiazine 3c , comprising a phenyl group at R, was higher compared to the one for 2H -1,4-benzothiazines with a methyl group or a hydrogen atom at R (Table 2 , entry 1–3). Negative controls of biotransformations of 2H -1,4-benzothiazines without IRED again showed no conversion, indicating that the utilized GDH has no side-activity toward this imine reduction. Furthermore, we found that IREDs catalyze the reduction of 2H -1,4-benzothiazines with high to excellent enantioselectivities (83–99% ee), and provided an access to both enantiomers of the 3,4-dihydro- 2H -1,4-benzothiazines with high enantiomeric excess (Table 2 , entry 2–3). Moreover, a higher enantioselectivity was observed for the more sterically demanding substrate 3c , comprising a phenyl group at R (with 99% ee), compared to the 2 H -1,4-benzothiazine 3b , comprising a methyl group at R (with up to 99% ee). The imine reductases IRED5, IRED28 and IRED29 [22] , [29] were identified as most suitable enzymes for the reduction of 2H -1,4-benzothiazine 3c bearing a phenyl group at R. Notably, in addition to all tested 3-thiazolines IRED8 [22] turned out to be able to catalyze also the reduction of 2H -1,4-benzothiazines 3a and 3c , thus representing an IRED being able to accept nearly all of the examined sulfur-containing heterocyclic imines. DFT studies Taking into account the different activities of IREDs for 3-thiazolines ( 1 ) and 2H -1,4-benzothiazines ( 3 ) with higher ones for the latter molecules, it is noteworthy that the (same) tendency is also observed for organocatalysts (being able to reduce 2H -1,4-benzothiazines ( 3 ) but not 3-thiazolines ( 1 ) (Supplementary Fig. 1 , and Supplementary Methods)). In addition, these findings are in accordance with observations of the Turner group, who found higher activities for six-membered rings compared to five-membered rings when examining the biocatalytic reduction of cyclic imines [20] , [23] . Therefore, we were interested in rationalizing this phenomena. Interestingly, both reduction methods are based on dihydropyridine moieties as reducing agents, namely the cofactor NADPH + H + and a Hantzsch ester, respectively. Therefore, we performed orientating DFT studies (B3LYP 6-311 + G**; for further details, see Supplementary Methods) with a dihydropyridine mimic in combination with a structurally minimized 3-thiazoline and 2H -1,4-benzothiazine, both of which were N-protonated. The barriers of activation associated with the transition states are 23 kcal/mol for the former (Fig. 6 a) and 19 kcal/mol for the latter (Fig. 6 b). Even though these gas-phase calculations are based on simplified (protonated) model systems, the higher barrier for the reduction of 3-thiazolines compared to the one for 2H -1,4-benzothiazines is in good agreement with the lower activities found for imine reductases, as well as with the lack of reactivity for organocatalysts when reducing 3-thiazolines. This trend was also confirmed by calculations with the SMD intrinsic solvation model, as similar differences in the free energies of activation were obtained with parameters for water (17 kcal/mol vs. 13 kcal/mol) and chloroform (20 kcal/mol vs. 15 kcal/mol). Fig. 6 DFT studies. Transition states obtained by DFT calculations for the reduction of the non-substituted protonated 3-thiazoline ( a ) and protonated 2 H -1,4-benzothiazine ( b ) by means of a dihydropyridine mimic as a reducing agent (Gibbs free energies of activation Δ G 298 K are given) Full size image Process development on 3-thiazoline reduction The positive results concerning IRED-catalyzed reduction of sulfur-containing heterocyclic imines motivated us to start a process development exemplified by the enantioselective reduction of 3-thiazoline 1f by means of IRED8 [22] (Fig. 7 a). Towards this end, in an analogy to our previous work [25] , [35] an E . coli whole-cell catalyst was designed, overexpressing the prioritized IRED8 and a glucose dehydrogenase from Bacillus subtilis for in situ-cofactor recycling. Both genes, encoding for IRED and GDH, respectively, have been inserted on different plasmids (Fig. 7 b). Preparative scale experiments (40 mL) were performed with a substrate concentration of 100 mM and a lyophilized whole-cell catalyst using a Titrino apparatus to adjust the pH at 7 (Fig. 7 c). We found that the reaction proceed smoothly also on preparative scale giving a very high conversion (99%) and enantioselectivity (99% ee for the S -enantiomer) within 30 h reaction time. After work up the desired 3-thiazolidine ( S )- 2f was isolated in 78% yield (Fig. 7 a). Fig. 7 Process development on 3-thiazoline reduction. a Whole-cell catalyzed reduction of 3-thiazoline 1f on 18 g L −1 scale, which corresponds to a substrate concentration of 100 mM. After 30 h of reaction time ( S )- 2f was obtained with 99% conversion (conv.) and 99% enantiomeric excess (ee) and was isolated with 78% yield. b Design of the recombinant whole-cell catalyst, containing imine reductase (IRED) from Mycobacterium smegmatis in a pET22b(+) vector and glucose dehydrogenase (GDH) from Bacillus subtilis in a pACYCDuet-1 vector. c Reaction setup for preparative scale experiment Full size image In summary, we reported a methodology which enables a reduction of 3-thiazolines under formation of the resulting 3-thiazolidines with high conversion and enantioselectivity of at least 96% ee and up to 99% ee, avoiding undesired ring-opening or other side reactions. This process technology, which is based on the use of IREDs as catalysts, has a broad substrate range and was also applied successfully to other sulfur-containing heterocyclic imines such as 2H -1,4-benzothiazines. Furthermore, the trends for the reduction of different substrates could be rationalized by molecular modeling and an initial process development was also conducted, demonstrating the suitability of this method for preparative use. In future work, the focus will be on rationalizing the enzymatic reaction course and the enantioselectivity of this process by means of molecular modeling. Biotransformations of 3-thiazolines Biotransformations of 3-thiazolines (which were synthesized as described in Supplementary Methods; related NMR data are shown in Supplementary Figs. 40 – 55 ) were performed on 10 mL scale at 30 °C and 500 r.p.m. 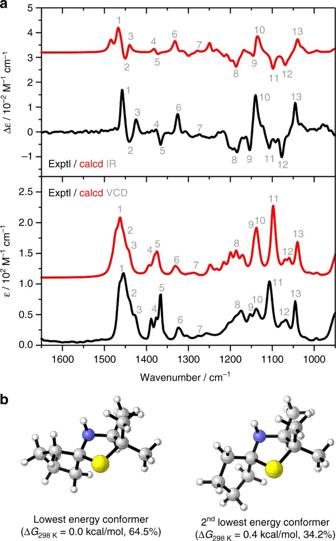Fig. 4 Determination of absolute configuration of2f.aComparison of the experimental and calculated IR and VCD spectra of (S)-2f(numbers indicate some characteristic band assignments).bStructures of the two main conformers of (S)-2f, corresponding relative Gibbs free energies ΔG298 Kand the corresponding Boltzmann weights in 100 mM KP i buffer pH 7, with 2% methanol as cosolvent containing 40 mM d -glucose, 20 mM 3-thiazoline 1a–f , 1.2 mg mL −1 (in case of substrate 1d and 1f and IRED8) or 5 mg mL −1 IRED crude extract (in the other cases shown in Table 1 , see Supplementary Table 4 , Supplementary Methods for codon-optimized gene sequences, protein sequences, Supplementary Figs. 8 – 38 for plasmid structures and Supplementary Fig. 39 for SDS-Page), 24 U (in case of 1.2 mg mL −1 IRED) or 100 U of GDH (in the other cases shown in Table 1 ) and 0.1 mM NADP + . After 24 h, the reaction was stopped by adding 200 µL of 32% NaOH solution and 10 mL of dichloromethane. Phase separation was promoted by centrifugation and the conversion was determined by analyzing the organic phase by means of achiral GC (Supplementary Figs. 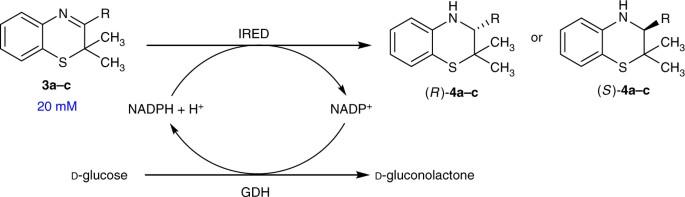Fig. 5 Imine reductase-catalyzed reduction of 2H-1,4-benzothiazines 56 – 60 , Supplementary Table 5 and Supplementary Methods; synthesis of racemic 3-thiazolidine reference compounds is described in Supplementary Methods and related NMR data are shown in Supplementary Figs. 61 – 70 ). For determination of the enantiomeric excess, samples were derivatized according to General Procedure 5 in the Supplementary Methods (NMR data of derivatized references are shown in Supplementary Figs. 71 – 78 ) and then analyzed by SFC-HPLC (Supplementary Figs. 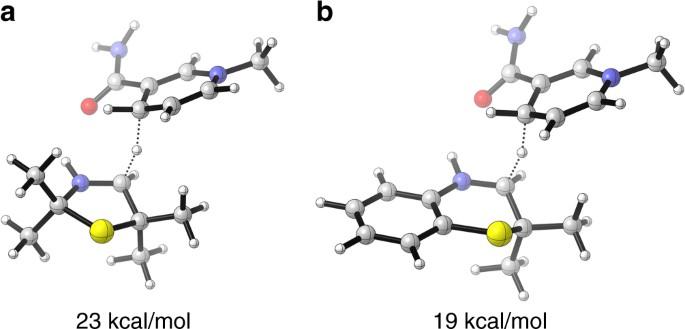Fig. 6 DFT studies. Transition states obtained by DFT calculations for the reduction of the non-substituted protonated 3-thiazoline (a) and protonated 2H-1,4-benzothiazine (b) by means of a dihydropyridine mimic as a reducing agent (Gibbs free energies of activation ΔG298 Kare given) 79 – 82 , Supplementary Table 6 and Supplementary Methods). The results of these experiments are shown in Table 1 , details about performing of negative controls are provided in the Supplementary Methods. The biotransformation on preparative scale (40 mL) using a whole-cell catalyst was performed in a similar fashion and is described in detail in Supplementary Methods. 1 H and 13 C NMR spectra of ( S )- 2f are shown in Supplementary Figs. 83 and 84 . Biotransformations of 2H-1,4-benzothiazines Biotransformations of 2H -1,4-benzothiazines (which were synthesized as described in Supplementary Methods; related NMR data are shown in Supplementary Figs. 40 – 43 and 85 – 92 ) were performed in a similar fashion as the biotransformations of 3-thiazolines. The conversion was determined by analyzing the organic phase by SFC-HPLC (Supplementary Figs. 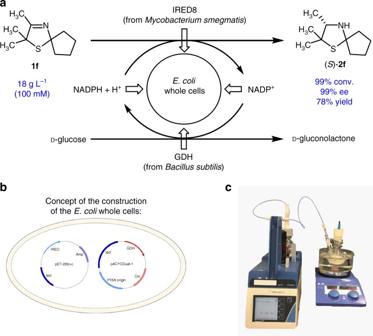Fig. 7 Process development on 3-thiazoline reduction.aWhole-cell catalyzed reduction of 3-thiazoline1fon 18 g L−1scale, which corresponds to a substrate concentration of 100 mM. After 30 h of reaction time (S)-2fwas obtained with 99% conversion (conv.) and 99% enantiomeric excess (ee) and was isolated with 78% yield.bDesign of the recombinant whole-cell catalyst, containing imine reductase (IRED) fromMycobacterium smegmatisin a pET22b(+) vector and glucose dehydrogenase (GDH) fromBacillus subtilisin a pACYCDuet-1 vector.cReaction setup for preparative scale experiment 93 – 95 , Supplementary Table 7 and Supplementary Methods; synthesis of racemic 3-3,4-dihydro-2 H -1,4-benzothiazine reference compounds is described in Supplementary Methods and related NMR data are shown in Supplementary Figs. 96 – 101 ). The results of these experiments are shown in Table 2 , details are provided in Supplementary Methods. Data availability The data that supports the findings of this study are available from the corresponding author upon request.